Coordination modulation of iridium single-atom catalyst maximizing water oxidation activity Single-atom catalysts (SACs) have attracted tremendous research interests in various energy-related fields because of their high activity, selectivity and 100% atom utilization. However, it is still a challenge to enhance the intrinsic and specific activity of SACs. Herein, we present an approach to fabricate a high surface distribution density of iridium (Ir) SAC on nickel-iron sulfide nanosheet arrays substrate (Ir 1 /NFS), which delivers a high water oxidation activity. The Ir 1 /NFS catalyst offers a low overpotential of ~170 mV at a current density of 10 mA cm −2 and a high turnover frequency of 9.85 s −1 at an overpotential of 300 mV in 1.0 M KOH solution. At the same time, the Ir 1 /NFS catalyst exhibits a high stability performance, reaching a lifespan up to 350 hours at a current density of 100 mA cm −2 . First-principles calculations reveal that the electronic structures of Ir atoms are significantly regulated by the sulfide substrate, endowing an energetically favorable reaction pathway. This work represents a promising strategy to fabricate high surface distribution density single-atom catalysts with high activity and durability for electrochemical water splitting. Electrochemical water splitting is considered as a sustainable option for large-scale hydrogen production by using renewable energy, such as solar, wind and hydropower [1] , [2] , [3] . However, the sluggish kinetics of water electrolysis results in high overpotentials for both hydrogen evolution reaction (HER) and oxygen evolution reaction (OER) [4] , [5] , thus significantly sacrificing the energy efficiency and increasing the hydrogen production cost [6] , [7] . Especially, the OER reaction involves a four-electron process which suffers from ten times higher overpotentials than that of HER, making it a bottleneck process in the overall water electrolysis system [4] , [8] . The commercial electrocatalysts used for water oxidaton in alkaline electrolyzer are Ni-based catalysts [9] . However, their catalytic performance remains far from satisfactory for the cost competiveness of hydrogen production. Thus, tremendous efforts have been made to improve the OER performance [10] , thus achieving high-efficiency electrolysis for cost-effective hydrogen energy in alkaline electrolyzer. So far, the catalysts for OER need to utilize precious metals, such as iridium (Ir) and ruthenium (Ru), to suppress the overpential during the water electrolysis process [11] . The utilization of precious metal catalysts significantly impairs the cost competitiveness of hydrogen production via electrochemical water splitting in comparison with other conventional hydrogen production technologies from the steam reforming process [12] , thus hindering the wide deployment of the electrolytic hydrogen production technology in the future [13] , [14] , [15] . Single-atom catalysts (SACs) provide a promising option to significantly reduce the utilization amount of precious metal catalysts by maximizing the atom-efficiency of precious metal elements in catalyst materials [16] , [17] , [18] , [19] , [20] , [21] . Recently, tremendous efforts have been devoted to developing efficient SACs for suppressing the OER overpotentials and improving the reaction kinetics for electrochemical water splitting [22] , [23] , [24] , [25] . It has been proved that the utilization of SACs could significantly improve the intrinsic activity of precious metal elements for the OER process and result in high mass activity [24] , [26] , [27] . The interaction between individual precious metal atoms and support substrate plays essential roles in modulating the microenvironment of active sites and consequently improves their activity and durability [28] , [29] , [30] . Various substrate materials have been attempted to maximize the mass activity of previous metals [31] , [32] , [33] , [34] , [35] . Despite these endeavors in developing suitable substrates for OER catalysts [17] , [36] , [37] , the fundamental understanding of the interaction between the substrate and the supported isolated atoms is still illusive [38] , [39] , [40] . Another major challenge in the fundamental science of SACs is to enhance the surface distribution density of active sites on the outer surface of substrates, rather than embedded inside the bulk materials [28] , [38] . Herein, we report a facile and scalable strategy to fabricate a low mass loading but high surface distribution density Ir SAC by anchoring on the Ni (3-x) Fe x S 2 (Ir 1 /NFS) nanosheet arrays via a two-step electrochemical method. The separation of substrate construction and Ir SAC deposition makes the distribution of Ir atoms only on the surface of the substrate, rather than inside the electrode, therefore maximizing the utilization of precious metals. As a result, the Ir 1 /NFS exhibits a high OER catalytic performance, which delivers an ultra-low overpotential of ~170 mV at a current density of 10 mA cm −2 with an ultra-high turnover frequency (TOF) of 9.85 s −1 at an overpotential of 300 mV. Density functional theory (DFT) calculations predict that the suitable chemical environment of Ir single-atom on the surface of NFS by Ir-S-M bond (M stands for Ni or Fe) efficiently reduces the kinetic energy barrier to form *OOH group from *O group, and thus accelerates the OER process. Catalysts fabrication and characterization The fabrication process of Ir 1 /NFS on a Ni foam electrode is illustrated in Fig. 1a . In order to separate the substrate construction and Ir SAC deposition processes, the nickel-iron sulfide nanosheets were firstly deposited on a Ni foam electrode by sweeping the potentials between 0.2 V and −1.2 V versus Hg/HgO reference electrode in a solution containing thiourea (TU) and nickel-iron precursors. Subsequently, the iridium precursor was added into the electrolyte and the electrode was swept between 0.3 V and −0.3 V versus Hg/HgO reference electrode for Ir single-atoms deposition (see details in experimental methods). As a result, the Ir atoms were deposited on the surface of NFS substrate, rather than inside the electrode, therefore maximizing the utilization of Ir atoms. Notably, thiourea plays an essential role in forming the sulfide substrate during the first deposition step and stabilizing the Ir precursor in the electrolyte during the second deposition step. Raman spectra shows a negative shift (~10 cm −1 ) for the peak at 489 cm −1 with increasing thiourea concentration (Supplementary Fig. 1 ), indicating that Ir ions form the complex of Ir(TU) x in the electrolyte [41] . The formation of complex ions prevents the formation of Ir clusters and nanoparticles during the deposition process. When without adding thiourea in the electrolyte, the Ir SAC on nickel-iron hydroxide substrate (Ir 1 /NFH) was formed after the same deposition procedure. Fig. 1: Electron microscope analysis of the Ir 1 /NFS. a Schematic illustration of the deposition to form the Ir 1 /NFS with two-step method. b TEM image of as-prepared the Ir 1 /NFS. Scale bar, 200 nm. c HAADF-STEM image of the Ir 1 /NFS (inset: SAED pattern) and the high density bright dots highlighted by yellow circles in an area of 5 nm × 5 nm. Scale bar, 5 nm. d HAADF image and the corresponding EDX elemental mappings of Ni, Fe, Ir, S, and O. Scale bar, 200 nm. Full size image The scanning electron microscopy (SEM) characterization results reveal that the Ir 1 /NFS catalyst displays a highly porous surface morphology with interconnected wrinkles (Supplementary Fig. 2 ), which is helpful to expose high surface area and render more active sites. The corresponding transmission electron microscope (TEM) image further confirms that the Ir 1 /NFS nanosheets are composed of a fluffy ultrathin layered structure (Fig. 1b ). The high-angle annular dark field-scanning transmission electron microscopy (HAADF-STEM) image reveals that the high-density isolated Ir atoms are homogeneously dispersed on the surface of NFS, without showing any aggregated clusters and nanoparticles (Fig. 1c , and Supplementary Fig. 3 ). The intensity line profile confirms that the Ir atom is located on the surface of NFS (Supplementary Fig. 4 ) [31] . Significantly, as shown in the framed area of Fig. 1c , the surface distribution density of Ir 1 atoms reaches up to ~3 atoms per square nanometer, which is higher than most of ever-reported SACs in literatures [16] , [17] , [23] . As shown in the inset of Fig. 1c , the selected area electron diffraction (SAED) pattern presents the diffraction spots for (110), (113), and (003) planes from a hexagonal structure of NFS nanosheets. The elemental mapping results based on the energy-dispersive X-ray (EDX) further prove that the Ir element is uniformly distributed on the NFS nanosheets in a large scale area without showing any aggregation phenomena (Fig. 1d ). Notably, the mass content of Ir in Ir 1 /NFS is determined to be ~0.6 wt% by the inductively coupled plasma mass spectrometry (ICP-MS) measurement. For comparison, the morphology and structure of Ir 1 /NFH were also characterized by using SEM and TEM. The electrode with Ir 1 /NFH also shows porous surface morphology similar to the electrode with Ir 1 /NFS (Supplementary Fig. 5 ). However, the Ir 1 /NFH catalyst possesses thicker nanosheets in comparison to the Ir 1 /NFS catalyst (Supplementary Fig. 6 ). The HAADF-STEM images reveal that the isolated Ir atoms are distributed on the NFH nanosheets, showing less aggregated Ir clusters (Supplementary Figs. 7 and 8 ). Furthermore, the corresponding EDX elemental mappings also show a homogeneous Ir distribution in the Ir 1 /NFH catalyst (Supplementary Fig. 9 ). Notably, the Ir mass loadings in Ir 1 /NFH is ~0.54 wt% by ICP-MS measurement, which is very close to the Ir loading in Ir 1 /NFS. Based on these characterization results, it indicates that the sulfide substrate is more favorable for forming high surface distribution density Ir single-atom in comparison with the hydroxide substrate. In order to prove this hypothesis, various precious metal SACs on NFS were fabricated following the same synthesis procedure, including Ru 1 /NFS, Au 1 /NFS, and Pt 1 /NFS (Supplementary Figs. 10 – 12 ). The isolated Pt 1 , Au 1 , and Ru 1 can be homogeneously dispersed on the surface of NFS, without showing any aggregated clusters and nanoparticles (Supplementary Figs. 13 – 15 ). The X-ray diffraction (XRD) patterns reveal that both Ir 1 /NFS and NFS possess the same crystalline structure that can be assigned to a crystal phase (PDF# 44-1418) of Ni 3 S 2 (Fig. 2a and Supplementary Fig. 16 ), indicating that the electrochemical process for Ir SAC deposition does not change the structure of NFS substrate. In contrast, the XRD patterns of both Ir 1 /NFH and NFH show less crystalline structure with two broad peaks at 35° and 62°, which can be assigned to a crystalline structure of Ni(OH) 2 ·0.75·H 2 O (PDF# 038-0715). X-ray photoelectron spectroscopy (XPS) was conducted to investigate the valence states of different elements in the catalysts. The core level Ir 4 f spectra of Ir 1 /NFS shows two peaks at 66.0 eV (Ir 4 f 5/2 ) and 62.9 eV (Ir 4 f 7/2 ), respectively. For comparison, the corresponding binding energy of Ir for Ir 1 /NFS is slightly lower than that for Ir 1 /NFH (63.2 eV for Ir 4 f 7/2 ), confirming the weaker chemical interaction in Ir 1 /NFS than that in Ir 1 /NFH (Fig. 2b ). To further investigate the valence state of Ir, the XPS measurements for IrCl 3 ·xH 2 O and IrO 2 were performed as references. It is observed that the valence state of Ir single-atoms in Ir 1 /NFS is slightly below the Ir (III) species in IrCl 3 ·xH 2 O, and is much lower than the Ir (IV) species in IrO 2 (Supplementary Figs. 17 and 18 ). XPS depth profiling spectra of Ir 3+ 4 f show that the peak intensity of Ir 3+ 4 f decreases along with the increase of sputtering time while the peak intensity of Ni 2+ 3 p has no obvious change, which indicates that the Ir SACs are located on the surface of NFS nanosheets (Supplementary Fig. 19 ). In addition, the high-resolution XPS S 2 p spectrum implies the formation of Ir-S-M (M stands for Ni or Fe) bond in Ir 1 /NFS, further confirming the charge transfer from Ir atoms to the substrate (Fig. 2c ). Notably, SO x 2− species are observed in the S 2 p spectra, indicating that the surface sulfur element is oxidized to some extent. The Ni 2+ 2 p and Fe 3+ 2 p XPS spectra of Ir 1 /NFS have no shift compared with that in NFS (Figs. 2d, e ). Moreover, we further studied the charge transfer between other SACs and the sulfide substrate, including Ru 1 /NFS, Au 1 /NFS, and Pt 1 /NFS. It is observed that the valence states of Ru, Au, and Pt in Ru 1 /NFS, Au 1 /NFS, and Pt 1 /NFS are Ru 3+ [463.3 eV (4 f 7/2 )], Au 3+ [83.9 eV (4 f 7/2 )], and Pt 4+ [72.8 eV (4 f 7/2 )] based on the XPS spectra (Supplementary Figs. 20 – 22 ), suggesting that the charge transfer also exist between various precious metal atoms and the NFS substrate. Fig. 2: Physicochemical property characterization. a XRD pattern of the Ir 1 /NFS and Ir 1 /NFH. b XPS spectra of Ir 4 f region with fitting curves for Ir 1 /NFS and Ir 1 /NFH. c – e XPS spectra of ( c ) S 2 p , ( d ) Ni 2 p , and ( e ) Fe 2 p regions with fitting curves for Ir 1 /NFS and NFS. Full size image Electrochemical oxygen evolution performance The electrocatalytic performances of the Ir 1 /NFS for OER were evaluated in 1.0 M KOH solution. All potentials were calibrated with respect to the reversible hydrogen electrode (RHE) (Supplementary Fig. 23 ). The commercial Ir/C (5 wt%) and IrO 2 catalysts were also tested as a benchmark value for OER activity. Remarkably, the OER overpotential for Ir 1 /NFS is observed down to ~170 mV for reaching a current density of 10 mA cm −2 , which is much lower than Ir 1 /NFH (~190 mV) and also the benchmark catalysts (Fig. 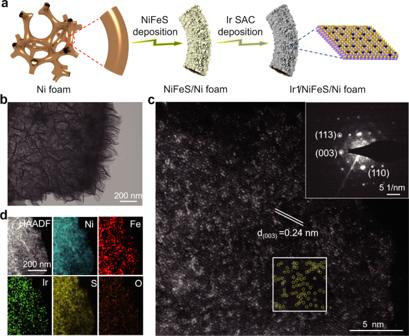Fig. 1: Electron microscope analysis of the Ir1/NFS. aSchematic illustration of the deposition to form the Ir1/NFS with two-step method.bTEM image of as-prepared the Ir1/NFS. Scale bar, 200 nm.cHAADF-STEM image of the Ir1/NFS (inset: SAED pattern) and the high density bright dots highlighted by yellow circles in an area of 5 nm × 5 nm. Scale bar, 5 nm.dHAADF image and the corresponding EDX elemental mappings of Ni, Fe, Ir, S, and O. Scale bar, 200 nm. 3a and Supplementary Table 1 ). Under more practical conditions, the OER overpotentials for Ir 1 /NFS are only 206 and 220 mV at current densities of 100 and 500 mA cm −2 , respectively. In contrast, the Ir 1 /NFH demonstrates much higher overpotentials of 234 and 257 mV, respectively. 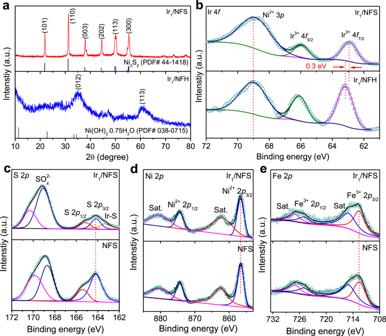Fig. 2: Physicochemical property characterization. aXRD pattern of the Ir1/NFS and Ir1/NFH.bXPS spectra of Ir 4fregion with fitting curves for Ir1/NFS and Ir1/NFH.c–eXPS spectra of (c) S 2p, (d) Ni 2p, and (e) Fe 2pregions with fitting curves for Ir1/NFS and NFS. We furthe investigated the substrate effect on the OER activity of Ir SAC by changing the ratio of Ni/Fe in the sulfide substrate (Supplementary Table 2 ). As shown in Supplementary Fig. 24 , the Ir 1 /Ni y Fe (6-y) S x (y = 0–6) electrodes have similar morphologies showing porous structures with interconnected wrinkles. The electrocatalytic activity of the Ni y Fe (6-y) S x (y = 0–6) substrate shows obvious Ni/Fe ratio dependence in 1.0 M KOH solution, among which the Ni 3 Fe 3 S x exhibits the superior performance (Supplementary Fig. 25 ). The Ir 1 /NFS catalysts also follow the similar activity trend when changing the Ni/Fe ratio of NFS substrate (Supplementary Figs. 26 and 27 ). Tafel plots provide further insights into the OER kinetics (Fig. 3b ). The Ir 1 /NFS has a very small Tafel slope (33 mV dec −1 ), which is lower than that of Ir 1 /NFH (35 mV dec −1 ), Ir/C (87 mV dec −1 ), and IrO 2 (95 mV dec −1 ). The low Tafel slope of Ir 1 /NFS suggests that the NFS substrate could significantly improve the electrochemical kinetics of Ir single-atoms. 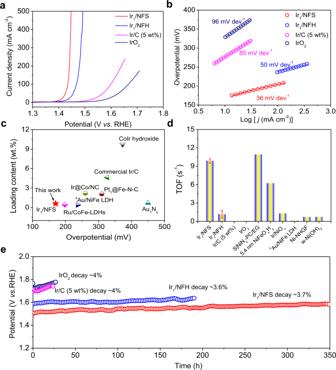Fig. 3: Electrochemical OER performance. aPolarization curves of Ir1/NFS, Ir1/NFH, Ir/C (5 wt%), and IrO2in 1.0 M KOH.bTafel plots derived from the polarization curves in (a).cThe comparison of overpotentials and precious metal loading contents in reported catalysts at a current density of 10 mA cm−2.dThe TOFs of state-of-the-art catalysts in alkaline solution (the error bars represent standard deviation values obtained from three independent measurements).eThe stability tests of Ir1/NFS, Ir1/NFH, Ir/C (5 wt%), and IrO2at 100 mA cm−2. Fig. 3: Electrochemical OER performance. a Polarization curves of Ir 1 /NFS, Ir 1 /NFH, Ir/C (5 wt%), and IrO 2 in 1.0 M KOH. b Tafel plots derived from the polarization curves in ( a ). c The comparison of overpotentials and precious metal loading contents in reported catalysts at a current density of 10 mA cm −2 . d The TOFs of state-of-the-art catalysts in alkaline solution (the error bars represent standard deviation values obtained from three independent measurements). e The stability tests of Ir 1 /NFS, Ir 1 /NFH, Ir/C (5 wt%), and IrO 2 at 100 mA cm −2 . Full size image In order to exclude the geometric effects on activity assessment, the OER activities of various catalysts were also tested on a flat Ni film (Ni/Au disc ), which was electrodeposited on a gold disc electrode. Ir 1 /NFS requires an overpotential of 230 mV for reaching a current density of 10 mA cm −2 on Ni/Au disc electrode, while Ir 1 /NFH (258 mV) need relatively high overpotential to deliver the same current density (Supplementary Fig. 28 ). Additionally, the specific activity of Ir 1 /NFS and Ir 1 /NFH were calculated based on the mass of Ir loadings on the Ni/Au disc electrode. The calculated specific activity for Ir 1 /NFS is 20.3 A g Ir −1 at 1.45 V versus RHE, which is ~1.55 times higher than that of Ir 1 /NFH (13.1 A g Ir −1 ). The specific activity of Ir 1 /NFS also outperforms most of the well-developed OER catalysts in literatures (Fig. 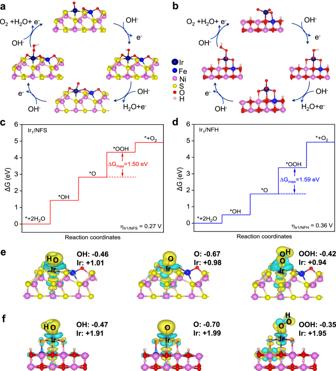Fig. 4: DFT theoretical models. a,bProposed 4e−mechanism of oxygen evolution reaction on Ir1/NFS and Ir1/NFH.c,dThe free energy profiles of four-step elementary reaction on Ir1/NFS and Ir1/NFH.e,fDiagrams of charge transfer between oxygen-containing intermediates and Ir atom during the oxygen evolution reaction of (e) Ir1/NFS and (f) Ir1/NFH. Green area represents the loss of electrons, while yellow area represents the opposite. 3c and Supplementary Table 4 ). The specific activity and turnover frequency (TOF) offers fundamental insights in evaluating the intrinsic activities of electrocatalysts [7] , [27] . The TOF was calculated based on the current density at the overpotential of 300 mV. The TOF of Ir 1 /NFS reaches up to 9.85 s −1 , which is an order of magnitude higher than that of Ir 1 /NFH (1.15 s −1 ) and previously reported values in literatures (Fig. 3d and Supplementary Table 5 ). The electrochemical impedance spectroscopy (EIS) was employed to investigate the charge transfer kinetics on various catalysts at an overpotential of 250 mV on Ni/Au disc . Besides the similar resistance of the electrolyte and electrode, the charge transfer resistance (R ct ) for Ir 1 /NFS (~26.5 Ω) is much lower than that for Ir 1 /NFH (~83.1 Ω) based on the fitted value according to the equivalent circuit (Supplementary Fig. 29 and Supplementary Table 6 ). Furthermore, the electrochemical double-layer capacitances (C dl ) was calculated to evaluate the electrochemically effective surface areas (ECSA) utilized a cyclic voltammetry method [42] , [43] . It is noted that the C dl of Ir 1 /NFS (3.7 mF cm −2 ) is ~2.0 times greater than that of the Ir 1 /NFH (1.3 mF cm −2 ), manifesting that Ir 1 /NFS possesses the most catalytic active sites for OER (Supplementary Fig. 30 ). The stability of catalyst is a critical parameter of OER performance, especially for practical applications. The chronoamperometry method was utilized to estimate the stability of Ir 1 /NFS and other samples at an overpotential of 250 mV on Ni foam electrodes. Strikingly, the Ir 1 /NFS displays a relatively higher and more stable current density (~50 mA cm −2 ) than that of Ir 1 /NFH (~27 mA cm −2 ) (Supplementary Fig. 31 ). Moreover, we evaluated the long-term electrochemical stability by using a chronopotentiometric technique at a relatively high current density of 100 mA cm −2 . Ir 1 /NFS demonstrates a superior stability performance, showing only ~3.7% of activity decay after 350 h, which is much better than Ir 1 /NFH (~3.6% decay after 198 h), Ir/C (5 wt%) (~4% decay after 25 h) and IrO 2 (~4% decay after 25 h) (Fig. 3e ). To further investigate the leaching effect of the catalyst after a long-term OER test (100 h at 100 mA cm −2 ), the amounts of dissolution elements from Ir 1 /NFS into the electrolyte was detected by ICP-MS measurement. As shown in Supplementary Fig. 32 , the Ir content in electrolyte for Ir 1 /NFS electrode is only ~1 ppb, indicating that the Ir element is stable in the Ir 1 /NFS catalyst during OER test. On the other hand, the Ni, Fe, and S content in electrolyte for Ir 1 /NFS electrode is determined to be ~5 ppb, ~13 ppb, and ~98 ppb, respectively, implying that the substrate transformation corrosion take place during the OER test. To further demonstrate the overall electrochemical water splitting, a large-area Ir 1 /NFS electrode (20 cm × 30 cm) was prepared (Supplementary Fig. 33 ), which was used to build up a two-electrode electrolysis device for water electrolysis. NiFe-OH-PO 4 was used as hydrogen evolution catalyst in this device which was synthesized according to the previous literature [44] . As shown in Supplementary Fig. 34 , the water electrolysis process could be driven by a single-cell AAA battery with a nominal voltage of ~1.5 V (Supplementary Movie 1 ). In addition, the morphology characterizations of the post-OER Ir 1 /NFS show that the initial nanosheet arrays with interconnected wrinkles are still maintained after testing for 10 h at an overpotential of 250 mV (Supplementary Fig. 35 ). The TEM images reveal that the post-OER Ir 1 /NFS nanosheets are composed of a fluffy ultrathin layered structure (Supplementary Fig. 36 ). The SAED patterns of the post-OER Ir 1 /NFS showed two diffraction rings, indicating an amorphous structure transformation after the OER test. The resulting EDX mapping images (Supplementary Fig. 37 ) show that Ni, Fe, Ir, S, and O are still homogeneously distributed over the entire post-OER Ir 1 /NFS sample. In addition, the HAADF-STEM images exhibit that the monoatomic Ir atoms (bright dots) uniform disperse on the surface of substrate and have no obvious aggregated clusters (Supplementary Figs. 38 and 39 ). Compared with the initial Ir 1 /NFS, the crystal structure post-OER Ir 1 /NFS shows a poor crystalline structure, but the main peaks of NFS can be detected as shown in Supplementary Fig. 40 . In addition, as shown in the Supplementary Fig. 41 , the Ir-S-M (M stands for Ni or Fe) bond is still maintained in the post-OER Ir 1 /NFS according to the S 2 p spectrum. It is noted that the binding energy of Ir 3+ 4 f 7/2 in post-OER Ir 1 /NFS has a negatively shift (~0.1 eV) compared with that in Ir 1 /NFS, indicating the coordination change occur during the OER test. The XPS spectra of S 2 p in post-OER Ir 1 /NFS show that the peak strength ratio of S 2− and SO x 2− displays some predictable changes, implying that the surface sulfur element of NFS is oxidized to some extent [45] , [46] , [47] . Mechanistic understanding on substrate effect on Ir SAC To further study the different OER activities on Ir 1 /NFS and Ir 1 /NFH structure models, the spin-polarized density functional theory calculations were employed to simulate the OER process based on the 4 e − mechanism proposed by Nørskov (Fig. 4a, b ) [48] , [49] . The Gibbs free energy profiles were calculated to investigate the nature of the activity difference between Ir 1 /NFS and Ir 1 /NFH and the free energy change of each elementary step is listed in Supplementary Table 7 . The rate-determining step towards OER for the loaded Ir atom is the conversion of *O to *OOH (Fig. 4c, d ), consistent with the previous studies under alkaline conditions [50] , [51] . In comparison with the limiting potential of 1.59 V versus computed hydrogen electrode (CHE) for Ir 1 /NFH’s rate-determining step, the loaded Ir atom on Ir 1 /NFS possesses a better activity with the significantly lower limiting potential of 1.50 V versus CHE. This result implies that the replacement of the substrate from oxide to sulfide can efficiently reduce the limiting potential and greatly enhance OER activity. As shown in Supplementary Figs. 43 and 44 , the additional theoretical analysis of the NFS without Ir SAC emphasizes that the Ir SAC is the main factor for the exceptional alkaline OER catalysis of the Ir 1 /NFS. Fig. 4: DFT theoretical models. a , b Proposed 4e − mechanism of oxygen evolution reaction on Ir 1 /NFS and Ir 1 /NFH. c , d The free energy profiles of four-step elementary reaction on Ir 1 /NFS and Ir 1 /NFH. e , f Diagrams of charge transfer between oxygen-containing intermediates and Ir atom during the oxygen evolution reaction of ( e ) Ir 1 /NFS and ( f ) Ir 1 /NFH. Green area represents the loss of electrons, while yellow area represents the opposite. Full size image Then we calculated the electronic properties of Ir atoms on different substrates to get more deep insights into the effect of substrate on the OER catalytic performance. To get more deep insights into the effect of substrate on the OER catalytic performance, we calculated the electronic properties of Ir atoms on different substrates. The total density of states (TDOS) (Supplementary Fig. 45 ) shows that Ir 1 /NFS has more electronic states near the Fermi level compared to Ir 1 /NFH, resulting in higher electrical conductivity, which is consistent with the results of resistance test. As the active site for adsorbing different intermediates, the electronic properties of the 4 d orbitals of the Ir atom are of concern to us. The projected density of states (PDOS) results (Supplementary Figs. 46 and 47 ) suggest that the electrons on Ir atoms in Ir 1 /NFS are closer to the Fermi level, and tend to be delocalized throughout the reaction compared with Ir 1 /NFH, which contributes to the enhanced electrochemical performance because of the elevated electron transfer. Furthermore, the differential charge density of the surface of Ir 1 /NFS and Ir 1 /NFH was adopted to rationalize the OER activity difference observed in the experiments. Combined with Bader charge analysis [52] , [53] , we have thoroughly studied the charge transfer between Ir atoms and different intermediates (Fig. 4e, f , and Supplementary Table 8 ). Compared with oxide substrates, Ir atoms on sulfide substrates tend to lose fewer electrons and exhibit a lower valence, which leads to the relatively weaker coupling of Ir atoms and oxygen-containing intermediates (Supplementary Table 9 ). There is still a linear relationship between the adsorption Gibbs free energy of intermediates *O and *OOH on Ir 1 /NFS (2.90 eV) and Ir 1 /NFH (2.86 eV). Charge transfer from substrate to form *O/Ir 1 from *OH/Ir 1 and the back transfer from *O/Ir 1 to form *OOH/Ir 1 is closer to each on Ir 1 /NFS than Ir 1 /NFH, which indicates that the replacement of the substrates is just conducive to the equal distribution of the reaction Gibbs free energies of the transfer from *OH to *O and *O to *OOH and lowers the rate-limiting potential. Meanwhile, we considered the oxidation of the substrate near iridium atoms to simulate the influence of the oxidizing environment (Supplementary Figs. 48 and 49 ). According to our results, the theoretical overpotential increased to varying degrees according to the number of oxygen atoms replaced. Comparing these overpotentials, conclusion can be drawn that the excellent catalytic activity exhibited by Ir 1 /NFS is closely related to the loading of iridium atoms on sulfur atoms. The oxidation of the substrate may destroy the chemical environment around the iridium atoms, which on the other hand demonstrates the superiority of the sulfide substrate. Therefore, both theoretical and experimental results are in agreement that the OER performance could be increased by dispersing Ir on NFS support with strong synergetic coupling which significantly enhanced intrinsic electrocatalytic activity and stability. In summary, the Ir 1 /NFS was synthesized via a general strategy to anchor a low mass loading but high distribution density Ir single-atom sites on the NFS support by a two-step electrochemical method. Compared with Ir 1 /NFH, Ir 1 /NFS reveals an excellent OER performance in alkaline electrolyte. Based on DFT calculations, the superior activity could be attributed to the Ir-S moiety in Ir 1 /NFS, manifested in favorable formation of the *OOH intermediate in the OER process. Meanwhile, the weak interaction between isolated Ir atoms and NFS is optimal to proceed OER compared with that Ir-O-M bond in Ir 1 /NFH, avoiding formation of the high oxidation state of Ir in Ir 1 /NFS. This work can help us understand the interaction of the sulfide substrate and precious metal single-atom catalysts for water oxidation, which may also inspire further work in catalyst design in the broad high concentration and stability of single atomic catalysis area. Synthesis of Ir 1 /NFS Ni foam (NF, thickness: 0.5 mm) was sonicated in 5.0 M HCl solution to remove surface oxide layer. Then, the Ni foam was washed with water and acetone, subsequently, dried at 40 °C under vacuum as electrode. Ni-modified gold electrode (Ni/Au disc ) was prepared by electrodeposition on Au electrode ( ϕ = 5 mm) in electrolyte containing 1.0 M NiSO 4 ·6H 2 O and 2.0 M Orthoboric acid at 60 °C. The current density of the prepared Ni/Au disc is 2.5 mA cm −2 for 1000 s under 600 rpm. A standard three-electrode electrochemical cell was used as the electrodeposition device which containing Ni foam and Ni/Au disc as the working electrodes, a carbon rod as the counter electrode and a Hg/HgO electrode (1.0 M KOH) as the reference electrode. Ir 1 /NFS electrode was prepared by a two-step electrodeposition method. The electrolyte was composed of 3 mM Ni(NO 3 ) 2 ·6H 2 O, 3 mM Fe(NO 3 ) 3 ·9H 2 O and 3 mM thiourea. The cyclic voltammetry (CV) was carried out in the potential range from 0.2 V to −1.2 V versus Hg/HgO at 5 mV s −1 for three cycles to get the NFS substrate. Then, 0.05 mM precursor (IrCl 3 ·xH 2 O) was added to the electrolyte and the potential range was changed to 0.3 V to −0.3 V versus Hg/HgO at 50 mV·s −1 for 15 cycles to get the Ir 1 /NFS. Besides Ni foam electrode, Ir 1 /NFS catalyst was also electrodeposited on Ni/Au disc following the same procedures. To verify the role of sulfide substrate, the Ir 1 /Ni y Fe (6-y) S x (y = 0–6) electrodes with a variable Ni/Fe ratio were prepared by adjusting the Ni and Fe ions concentration in the electrodeposited electrolytes. The electrodeposition was followed by the same procedures as the Ir 1 /NFS electrode fabrication. Synthesis of M 1 /NFS (M = Pt, Au, Ru) For the synthesis of Pt 1 /NFS, Au 1 /NFS, and Ru 1 /NFS, the precious precursors (H 2 PtCl 6 ·6H 2 O, HAuCl 4 ·4H 2 O, and RuCl 3 ·xH 2 O) replaced IrCl 3 ·xH 2 O in the electrolyte, respectively. The electrodeposition procedures were the same as these for the synthesis of Ir 1 /NFS. Synthesis of Ir 1 /NFH For the synthesis of Ir 1 /NFH, thiourea was removed from the electrolyte and the electrodeposition procedures were the same as these for the synthesis of Ir 1 /NFS. Prepared the Ir/C and IrO 2 electrodes To prepare the Ir/C ink, 11 mg of Ir/C (5 wt% of Ir, Premetek Co.) was dispersed in 1 ml of water and ethanol solution (1:4, v/v), followed by the addition of 45 μl of Nafion 117 solution (Sigma-Aldrich). The mixture was then magnetic stirred to form a homogenous ink. Meanwhile, the IrO 2 ink was also prepared, namely 5.14 mg of IrO 2 and 5 mg of Ketjen Black dispersed in 1 ml of water and ethanol solution (1:4, v/v), followed by the addition of 40 μl of Nafion 117 solution (Sigma-Aldrich). The mixture was then sonicated briefly to form a homogenous ink. The ink was drop-casted onto the Ni foam and Ni/Au disc electrodes and left dried in air. Characterizations The morphologies and structures of as-prepared samples were characterized by field-emission scanning electron microscopy (SEM, Hitachi, SU8010, 10 kV) and transmission electron microscopy (TEM, Hitachi, H7700, 100 kV). HAADF-STEM images, and energy-dispersive X-ray (EDX) mappings were obtained by using a JEOL, JEM − 2100, 200 kV. X-ray diffraction (XRD) patterns were measured by using a Bruker D8 Advance X-ray diffractometer equipped with Cu Kα radiation (λ = 1.5418 Å). X-ray photoelectron spectra (XPS) were performed by using a Thermo Scientific ESCALAB 250Xi with monochromatic Al Kα X-ray sources (1486.6 eV) at 2.0 kV and 20 mA. Inductively coupled plasma mass spectrometer (ICP-MS) was performed on iCAP 7400. Raman spectra was carried out on a Renishaw RM 3000 Micro-Raman system. Electrochemical characterization All electrochemical measurements were carried out with a three-electrode on the CHI 760E electrochemical workstation. As-prepared Ir 1 /NFS and Ir 1 /NFH electrodeposited on Ni foam (1 cm × 1 cm) and Ni/Au disc electrodes were used directly as the working electrode without any further treatments. A carbon rod was used as the counter electrode and a Hg/HgO electrode (1.0 M KOH) was used as the reference electrode in 1.0 M KOH solution. All potential values in electrochemical measurements were calibrated with respect to the reversible hydrogen electrode (RHE). The calibration was performed in the high purity hydrogen 1.0 M KOH electrolyte with a Pt wire as the working electrode and a carbon rod as the counter electrode. The measured potentials versus Hg/HgO were converted to the values with reference to a RHE using the following equation [54] , 
    E_RHE=E_Hg/HgO+0.197 V
 (1) Catalytic activity was assessed by linear sweep voltammetry (LSV) with a sweep rate of 5 mV·s −1 with 95% iR compensation. Tafel slopes were derived from the OER polarization curves obtained at 5 mV·s −1 . For iR compensation, an iR compensation level of 95% was applied by using the automated iR -correction function of the potentiostat [55] . Electrochemical impedance spectroscopy (EIS) curves were recorded under amplitude 5 mV, and the frequency ranged from 10 K Hz to 0.1 Hz at an overpotential of 250 mV. The Double-layer capacitance (C dl ) was determined by measuring the capacitive current associated with double-layer at non-Faradaic potential range charging from the scan-rate dependence of CV [43] . C dl was estimated by plotting the half of the difference of the anodic and cathodic current density against the scan rate. All chronopotentiometry and chronoamperometry measurements were conducted under the same experimental setup without iR compensation. Overall water splitting test condition: a two-electrode electrolysis device was fabricated by using Ir 1 /NFS as the OER catalyst and NiFe-OH-PO 4 as hydrogen evolution catalyst in 1.0 M KOH solution. The NiFe-OH-PO 4 was electrodeposited onto the Ni foam by CV in electrolyte containing 3.0 mM NiCl 2 ·6H 2 O, 3.0 mM FeCl 2 ·4H 2 O, and 1.0 mM NaH 2 PO 2 . The CV curves were carried out in the potential range from 0.2 V to −1.2 V versus Hg/HgO at 5 mV s −1 for three cycles to get the NiFe-OH-PO 4 catalyst. Subsequently, the Ir 1 /NFS and NiFe-OH-PO 4 catalysts were assembled into a two-electrode system, and the electrodes area were 2 cm × 2 cm, respectively. The overall water splitting was driven by a single-cell AAA battery with a nominal voltage of ~1.5 V in 1.0 M KOH. Calculation of turnover frequency (TOF) The TOF values of Ir 1 /NFS, and Ir 1 /NFH coated on Ni/Au disc were calculated according to the equation [56] , 
    TOF=j×A/4× F× m
 (2) where j is the current density obtained at overpotential of 300 mV in A cm −2 , and the contribution of the Ni and Fe active sites to the current density is deducted. A is the surface area of the Ni/Au disc electrode (0.19625 cm 2 ), F is the Faraday efficiency (96,485 C mol −1 ) and m is the number of moles of the Ir deposited onto the Ni/Au disc electrode which was calculated by ICP-MS measurement. Theoretical calculations In this study, all the spin-polarized calculations were performed by using the Vienna Ab-initio Simulation Package (VASP) with the projector augmented wave method for the core region and a plane-wave kinetic energy cutoff of 400 eV [57] , [58] , [59] . The DFT + U calculations were performed in calculating the nickel oxide system, while the value of U was 4.3 for Fe and 3.8 for Ni according to the previous studies [60] . The generalized gradient approximation method with Perdew-Burke-Ernzerh of (PBE) functional for the exchange-correlation term was used [61] . The models we adopted for calculation were modified from the surface of Ni 3 S 2 (003) [62] and Ni(OH) 2 (012), which are based on XRD and SADE results. After replacing the Ni atom with a Fe atom at the outermost layer, an Ir atom was loaded on S atoms or O atoms near it. In order to simulate the environment where oxygen is enriched on the electrode surface in actual electrocatalytic process, both Ir and Fe atoms have been highly coordinated by O atoms as shown in Fig. 4a and Supplementary Fig. 42 . Ir 1 /NFS model used in our calculation consists of 12.21 Å × 12.21 Å × 25.18 Å and Ir 1 /NFH consists of 9.31 Å × 1.93 Å × 22.06 Å. The large vacuum region was set at least 15 Å in z direction for the isolation of surface to prevent the interaction between two periodic units. A 3 × 3 × 1 Monkhorst-Pack sampled k-point grid was used to sample the reciprocal space. For the structure optimization, the convergence of energy and forces on each atom were set to be less than 1 × 10 −5 eV and 0.02 eV/Å. During our calculation, top two layers were fully relaxed and the other layers are fixed at the lattice positions. According to the OER cycle proposed by Nørskov [49] , the OER reaction follows the four-electron mechanism, corresponding to the four primitive steps listed in Eqs. ( 3 ) to ( 6 ), which involve adsorbed OH, O, and OOH intermediates on the surface (*), 
    ∗ +OH^-→∗OH+e^-
 (3) 
    ∗OH+OH^-→H_2O+∗O+e^-
 (4) 
    ∗O+OH^-→∗OOH+e^-
 (5) 
    ∗OOH+OH^-→O_2+H_2O+e^-
 (6) The Gibbs free energy changes for these four elemental steps can be expressed respectively as [48] , 
    G_1=μ_∗OH-μ_∗-(μ_OH^--μ_e^-)
 (7) 
    G_2=μ_∗O-μ_∗OH+μ_H_2O(l)-(μ_OH^--μ_e^-)
 (8) 
    G_3=μ_∗OOH-μ_∗O-(μ_OH^--μ_e^-)
 (9) 
    G_4=μ_∗+μ_H_2O(l)+μ_O_2(g)-μ_∗OOH-(μ_OH^--μ_e^-)
 (10) where \(\mu\) represents the chemical potentials of the indicated species. Here, the difference of the chemical potentials of the \({{OH}}^{-}\) species and the electron can be described as, 
    μ_OH^--μ_e^-=μ_H_2O(l)-(μ_H^++μ_e^-)
 (11) Meanwhile, the chemical potential of the proton and electron is related to that of H 2 according to the computational hydrogen electrode (CHE) approach. μ_H^++μ_e^-=1/2μ_H_2(g)-eU_RHE
 (12) where \({U}_{{RHE}}\) was the potential of the electrode relative to the RHE. Thus, Eqs. ( 13 )–( 16 ) can be rewritten as, 
    G_1=μ_∗OH-μ_∗-μ_H_2O(l)+1/2μ_H_2(g)-eU_RHE
 (13) 
    G_2=μ_∗O-μ_∗OH-μ_H_2O(l)+1/2μ_H_2(g)-eU_RHE
 (14) 
    G_3=μ_∗OOH-μ_∗O-μ_H_2O(l)+1/2μ_H_2(g)-eU_RHE
 (15) 
    G_4=μ_∗-μ_∗OOH+μ_O_2(g)+1/2μ_H_2(g)-eU_RHE
 (16) The chemical potential \(\mu\) was defined as [63] \(\mu =E+{ZPE}-T\times S\) , where E , ZPE , T , and S represented the total energy obtained from DFT calculations, the zero-point energy ( ZPE ), the temperature (298.15 K), the entropy obtained from vibrational frequency calculations, respectively. The entropies of gas-phase H 2 , and H 2 O were obtained from the NIST database (Computational Chemistry Comparison and Benchmark Database. http://cccbdb.nist.gov/ ) with standard condition. Due to the non-negligible error in the first-principles calculation, the chemical potential of oxygen molecule is calculated as \({\mu }_{{O}_{2}}=2{G}_{{H}_{2}O(l)}-2{G}_{{H}_{2}}+4.92{eV}\) . Then entropies of adsorbed species are considered according to vibrational entropy ( \({S}_{v}\) ) formula, 
    S_v=∑_iR{hv_i/k_BT[exp(hv_i/k_BT)-1]^-1-ln[1-exp(-hv_i/k_BT)]}
 (17) All the real vibrational frequencies of the surface-adsorbing species were included to calculate the correction of the free energy. Under ideal conditions, the OER reaction with a total energy change of 4.92 eV can be driven at 1.23 V, while the \(\triangle\) G of each elementary reaction would be equally divided into 1.23 eV. Therefore, the overpotential η is introduced to represent additional required potential and measure the catalytic activity of materials, which is defined in theoretical calculations as, 
    η =max[G_1,G_2,G_3,G_4]/e-1.23V
 (18)